The dynamic stator stalk of rotary ATPases Rotary ATPases couple ATP hydrolysis/synthesis with proton translocation across biological membranes and so are central components of the biological energy conversion machinery. Their peripheral stalks are essential components that counteract torque generated by rotation of the central stalk during ATP synthesis or hydrolysis. Here we present a 2.25-Å resolution crystal structure of the peripheral stalk from Thermus thermophilus A-type ATPase/synthase. We identify bending and twisting motions inherent within the structure that accommodate and complement a radial wobbling of the ATPase headgroup as it progresses through its catalytic cycles, while still retaining azimuthal stiffness necessary to counteract rotation of the central stalk. The conformational freedom of the peripheral stalk is dictated by its unusual right-handed coiled-coil architecture, which is in principle conserved across all rotary ATPases. In context of the intact enzyme, the dynamics of the peripheral stalks provides a potential mechanism for cooperativity between distant parts of rotary ATPases. Rotary ATPases are multi-subunit biological machines that couple proton (or occasionally sodium) translocation across membranes with ATP synthesis or hydrolysis [1] . Three evolutionarily related subtypes of rotary ATPases (F-, V- and A-type) are distinguished on the basis of their function and taxonomic origin [2] . F-ATPases, better known as F 1 F o ATP synthases, couple proton flow across membranes with ATP synthesis [3] . In contrast, eukaryotic vacuolar or V-ATPases operate in reverse, actively pumping protons across membranes using energy derived from ATP hydrolysis [4] . Eukaryotes contain both F- and V-ATPases, each highly specialized in its physiological function, but many prokaryotes contain only one of these complexes that can operate in either direction [5] , [6] . All sequenced archaea contain A-type ATPase/synthase complexes that are evolutionary closer to V-ATPases, but function primarily as ATP synthases [2] . The majority of eubacteria have F-type ATPases, but some, including T. thermophilus , contain an A-type ATPase (also called bacterial V-type ATPase) [7] . All rotary ATPases have a conserved architecture based on a water-soluble ATPase-active F 1 , V 1 or A 1 domain and a membrane-bound proton-translocating F o , V o or A o domain [1] , [8] . The A 1 domain of T. thermophilus has a catalytic head that contains a trimer of nucleotide-binding subunit A–B dimers and a central stalk composed of subunits D and F ( Fig. 1 ) [7] , [9] . The proton-translocating A o domain contains subunit C, together with a ring of 12 proteolipids (subunit L) and a single copy of the amphipathic subunit I that is located adjacent to the ring [10] , [11] . The proton channel is formed at the interface between the transmembrane portion of subunit I and the L-ring [12] . ATP synthesis and hydrolysis are coupled to proton translocation through rotation of the central stalk and L-ring relative to the nucleotide-binding domain and subunit I. An additional stator component is required to counteract the torque generated by the rotation of the central stalk and to connect the non-rotating nucleotide-binding subunits with subunit I. This essential component, known as the peripheral stalk or stator stalk, has recently become recognized as a hallmark of rotary ATPase taxonomy: F-type ATPases contain only one peripheral stalk [13] , [14] , [15] , [16] , A-type ATPases contain two [17] , [18] , [19] and eukaryotic V-type ATPases contain three [20] , [21] , [22] , [23] . Each of the A- and V-type peripheral stalks are composed of a heterodimer of subunits E and G [18] , [20] , [24] , whereas the subunit composition of the single F-type ATPase peripheral stalk is different [25] . 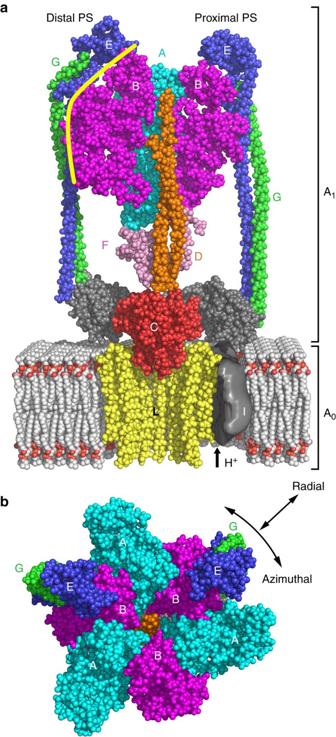Figure 1: Model of the intact A-ATPase obtained by fitting individual structures into the EM density of the intactT. thermophiluscomplex. (a) Side view: subunit A is shown in cyan, B in magenta, C in red, D in orange, F in pink, L in yellow, E in blue, G in green and soluble I in grey. Two A subunits and one B subunit were omitted for clarity. As there is currently no structure for the L-ring available in the protein data bank, we modified the theoretical model of a NMR-derivedE. colic12-ring (pdb entry: 1c17) to give a symmetrical c12-ring. The unknown structure of the transmembrane portion of subunit I is indicated by a cut-out EM density in grey, with the proton path indicated by an arrow. (b) Top view: Explanation of the definitions of 'radial' and 'azimuthal' as used in the text. PDB codes of coordinates used are: 3a5d:T. thermophilus(AB)3DF complex9, 1r5z:T. thermophilussubunit C58, 3k5b:T. thermophilusEG complex (PS1)26, 3rrk:Myotis rubersoluble I59and 1c17:E. colisubunit c12-ring model60. Figure 1: Model of the intact A-ATPase obtained by fitting individual structures into the EM density of the intact T. thermophilus complex. ( a ) Side view: subunit A is shown in cyan, B in magenta, C in red, D in orange, F in pink, L in yellow, E in blue, G in green and soluble I in grey. Two A subunits and one B subunit were omitted for clarity. As there is currently no structure for the L-ring available in the protein data bank, we modified the theoretical model of a NMR-derived E. coli c 12 -ring (pdb entry: 1c17) to give a symmetrical c 12 -ring. The unknown structure of the transmembrane portion of subunit I is indicated by a cut-out EM density in grey, with the proton path indicated by an arrow. ( b ) Top view: Explanation of the definitions of 'radial' and 'azimuthal' as used in the text. PDB codes of coordinates used are: 3a5d: T. thermophilus (AB) 3 DF complex [9] , 1r5z: T. thermophilus subunit C [58] , 3k5b: T. thermophilus EG complex (PS1) [26] , 3rrk: Myotis ruber soluble I [59] and 1c17: E. coli subunit c 12 -ring model [60] . Full size image The 3.1-Å resolution crystal structure of the T. thermophilus A-ATPase peripheral stalk [26] (hereafter referred to as PS1) showed that the overall architecture of the heterodimeric peripheral stalk consists of a globular head mainly made of the C-terminus of subunit E and a 120-Å long tail made of a right-handed parallel coiled-coil consisting of subunit G and the N-terminus of subunit E. Docking of this structure into a 23-Å resolution electron microscopy (EM) three-dimensional (3D) reconstruction of the intact A-ATPase [10] highlighted an apparent asymmetry between the two peripheral stalks, suggesting that these structures undergo conformational changes complementing the asymmetry of the nucleotide-binding subunits during the rotary catalytic cycle. Although the PS1 structure accounts reasonably well for the EM density at the distal stator site with reference to the ion channel, it fits the proximal site less well [26] . Docking of all remaining available X-ray structures into the 3D EM reconstruction of the intact T. thermophilus A-ATPase has provided us with a composite model of the intact complex ( Fig. 1 ) [26] . In this model, the central axis through the catalytic (AB) 3 assembly is not coincident with the central axis through the proteolipid ring, and hence the transmembrane domain is inclined to the catalytic domain ( Fig. 2 ). This tilt of the catalytic head relative to the transmembrane domain has also been observed in crystal structures of F-ATPase complexes ( Supplementary Fig. S1 ) [27] , [28] , [29] , [30] and in EM class averages of intact rotary ATPases that are free from crystal-packing forces [10] , [12] , [17] , [31] . In this arrangement, the transmembrane rings would make an eccentric (precession) movement relative to the fixed catalytic heads as the central stalk rotates [32] ( Supplementary Movies 1–4 ). However, in vivo , the proteolipid rings are inserted into the membrane and so the rotation axis will be fixed perpendicular to the plane of the membrane. Consequently, the catalytic domains will 'wobble' back and forth, changing their radial but not their azimuthal position (that is, the position along the circumference of the complex, Fig. 1b ), as the central stalk rotates ( Supplementary Movie 5 ). Hence, it is crucial for the peripheral stalks to be able to accommodate this wobbling movement of the catalytic head, while simultaneously counteracting the torque generated by rotation of the central stalk in an azimuthal direction. 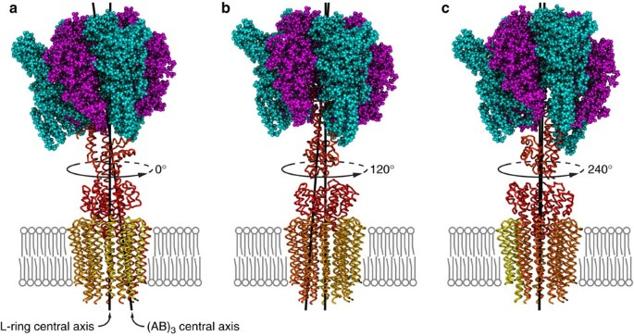Figure 2: The three rotational states of the composite model of theT. thermophilusA-ATPase. The central rotor (subunits D, F, C and the L-ring) is rotated by 0° (a), 120° (b) and 240° (c) about the central axis through the L-ring (as indicated) relative to the (AB)3ring. The central axis through the centre of the (AB)3ring is inclined with respect to the central axis through the L-ring (∼6° tilt). Figure 2: The three rotational states of the composite model of the T. thermophilus A-ATPase. The central rotor (subunits D, F, C and the L-ring) is rotated by 0° ( a ), 120° ( b ) and 240° ( c ) about the central axis through the L-ring (as indicated) relative to the (AB) 3 ring. The central axis through the centre of the (AB) 3 ring is inclined with respect to the central axis through the L-ring ( ∼ 6° tilt). Full size image Here, we provide a model of how the peripheral stalks are able to accommodate these structural requirements. We present the crystal structure of the T. thermophilus A-ATPase peripheral stalk (referred to as PS2) in a different conformation to that of PS1, obtained from an alternate crystal form [26] . Comparison of PS1 and PS2 structures in combination with conformations seen in EM reconstructions and with normal mode analyses (NMA) shows how the conformation of the peripheral stalk changes to complement the wobbling of the catalytic head during rotary catalysis. Furthermore, we show how the unusual right-handed coiled-coil structure of the peripheral stalk's tail can accommodate radial movements of the catalytic domain while constraining its azimuthal motions to counteract rotation of the central stalk. Rotary ATPases 'wobble' during their catalytic cycles All available crystal structures of A-ATPase subunits were docked into a 23-Å resolution 3D EM reconstruction of the T. thermophilus A-ATPase [10] resulting in a pseudo-atomic model of the intact complex that lacks only the ion channel-forming domain of subunit I, for which no structural information is available ( Fig. 1 ). In this model, the rotation axis of the central rotor is not coincident with the central axis through the catalytic head, and hence the central stalk protrudes at an angle from the catalytic domain leading to an inclination of the catalytic to the transmembrane domain ( Fig. 2 ). The same is true for available crystal structures of mitochondrial F 1 c n complexes ( Supplementary Fig. S1 ) [27] , [28] , [29] , [30] and it was noted previously that the central rotor in the yeast mitochondrial F 1 c 10 crystal structure would make an eccentric movement during rotation [32] . More recently, a single molecule analysis of the F 1 motor has identified a tilting of the central stalk induced by ATP binding [33] . Here, we have extended these analyses to define the extent of the movement in both types of rotary ATPases more precisely; geometric analysis gave an average angle of inclination of about 7° for both A- and F-ATPases ( Supplementary Figs S1, S2; Table 1 ). Table 1 Angles between central axis of proteolipid ring (F O /A O ) and central axis of catalytic headgroup (F 1 /A 1 ). Full size table Although the structures of A- and F-ATPases represent static views of dynamic molecular rotary motors, they enable estimation of the likely structural changes that are generated as rotation of the central stalk drives transitions between different nucleotide states. Insertion of the complex in the membrane will likely lead to the centre of rotation coinciding with the centre of the proteolipid ring, leading to a wobble of the catalytic head rather than an eccentric rotation of the proteolipid ring. To obtain the relative positions of the A-ATPase B subunits (to which the peripheral stalk predominantly binds), the atomic model was superposed upon itself using 120° and 240° rotations of the L-ring. These superpositions illustrate how the catalytic head wobbles on its axis as the central stalk rotates ( Fig. 2 ; Supplementary Movie 5 ), with the radial position of subunit B relative to the central rotation axis varying significantly, coupled with a change in the tilt of the catalytic head as the central stalk rotates. To preserve the interface between the peripheral stalks and subunit B (yellow line in Fig. 1a ), the peripheral stalk must be sufficiently flexible in this region to accommodate the wobbling of the catalytic head generated by the tilt of the central stalk. Crystal structure of PS2 and comparison with PS1 The overall architecture of the peripheral stalk consists of a C-terminal globular head, mainly made of subunit E, and an N-terminal, 120-Å-long heterodimeric right-handed coiled-coil, made of subunit G and the N-terminus of subunit E [26] . The unique right-handed coiled-coil nature of the complex results in almost parallel coils at the N-termini. Within the intact complex these are situated close to the membrane, where the interactions with the soluble domain of subunit I occur, whereas the C-terminal globular head is attached to the top of the nucleotide-binding domain distal to the membrane. Here, we present the structure of a peripheral stalk from a different crystal form (PS2) with a distinctly different conformation to PS1, determined to 2.25-Å resolution using multiple isomorphous replacement with anomalous scattering (MIRAS) from two heavy-atom derivatives (data collection and refinement statistics are given in Table 2 ). As in the PS1 crystal form, there are two heterodimers of subunit E and G per asymmetric unit that have very similar conformations with a root mean square deviation (RMSD) of 0.86 Å, yet the conformations of PS1 and PS2 differ significantly. Although the overall RMSD is only 3.1 Å between PS1 and PS2, and the secondary structure and inter-subunit contacts between subunits E and G are largely retained, there are two substantial conformational differences ( Fig. 3 ). First, a flexion of the long helices accentuates the concavity of the PS2 right-handed coiled-coil tail and, second, the globular head twists about the axis of the long helices. Superposition of the globular heads of PS1 and PS2 (using residues 100 to 188 of subunit E) thus leads to a maximum displacement of the tails by 28 Å. Table 2 Data collection and refinement statistics. 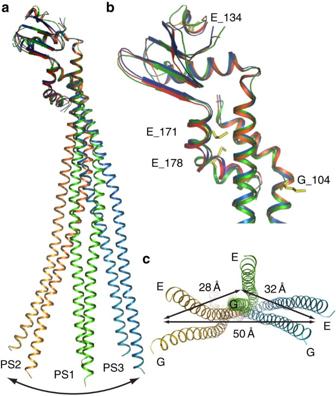Figure 3: Comparison of peripheral stalk structures. PS1, PS2 and PS3 were superposed by their globular domains (using residues 100–188 of subunit E). PS126is shown in green, PS2 in yellow to red colours and PS3 is shown in blue. (a) View from side, with black arrow representing maximum flexion between PS2 and PS3. The tail flexes primarily in a plane corresponding to a radial direction in the intact A-ATPase. (b) Superposition of peripheral stalk globular heads, with methionines present in PS1 highlighted in yellow and labelled, and (c) view from bottom, with black arrows indicating maximum displacement of helices. Full size table Figure 3: Comparison of peripheral stalk structures. PS1, PS2 and PS3 were superposed by their globular domains (using residues 100–188 of subunit E). PS1 [26] is shown in green, PS2 in yellow to red colours and PS3 is shown in blue. ( a ) View from side, with black arrow representing maximum flexion between PS2 and PS3. The tail flexes primarily in a plane corresponding to a radial direction in the intact A-ATPase. ( b ) Superposition of peripheral stalk globular heads, with methionines present in PS1 highlighted in yellow and labelled, and ( c ) view from bottom, with black arrows indicating maximum displacement of helices. Full size image Fitting PS1 and PS2 crystal structures into the EM density The conformation of PS1 is consistent with the electron density of the distal peripheral stalk from the 23-Å resolution 3D EM reconstruction of the intact A-ATPase [10] . However, neither PS1 nor PS2 structures fit into the EM density of the proximal peripheral stalk, indicating that neither crystal structure accounts for its conformation. To determine a putative conformation of the proximal peripheral stalk, we used molecular dynamics flexible fitting (MDFF) implemented in the NAMD2 package [34] to fit both the PS1 and PS2 crystal structures into the EM density ( Supplementary Movie 6 ). Both structures morph into essentially the same conformation, referred to as PS3, with a substantially improved fit into the EM density of the proximal peripheral stalk as reflected in a cross-correlation coefficient [35] of 0.92 compared with 0.86 and 0.83 for PS1 and PS2, respectively ( Supplementary Fig. S2 ). A superposition of the globular head domains of PS1, 2 and 3 shows how these three models relate to one another by a flexion of the right-handed coiled-coil tail and a swivel of the globular head ( Fig. 3 ). Notably, the conformational change from PS1 to PS3 is on the same trajectory as that from PS1 to PS2, albeit in the opposite direction, thus indicating that the same torsion angles are used. Peripheral stalk movements in context of the intact A-ATPase To simulate the movement of the peripheral stalks within the intact complex, all three peripheral stalk structures were docked into the pseudo-atomic model of the rotating intact complex. Again, we first simulated rotation of the central stalk while keeping the catalytic head fixed, which leads to an eccentric rotation of the L-ring ( Supplementary Movies 7–8 ). Intriguingly, the movement of the peripheral stalk structures follows the precession movement of the L-ring closely. This is remarkable given the crystal structures of PS1 and PS2 were derived from protein expressed and crystallized in the absence of the intact complex, indicating that the flexibility is inherent within the sequences of the peripheral stalk subunits. In the more physiological scenario, where the rotation axis of the transmembrane L-ring remains fixed perpendicular to the membrane, the different conformations of the peripheral stalk structures provide a similar mechanism by which the peripheral stalk can complement the wobbling of the catalytic head. Thus, the radial movement of the catalytic domain can be accommodated by the flexing of the right-handed coiled-coil while the tilting of the catalytic domain can be accommodated by the swivelling of the globular head ( Supplementary Movie 9 ). Normal mode analysis of peripheral stalk dynamics To further test this hypothesis, the conformational changes required to interconvert between the three peripheral stalk structures were modelled using NMA. NMA calculates vibrational modes and protein flexibility, and therefore helps to describe possible motions. For the analysis, atoms are modelled as point masses connected by springs, which represent the interatomic forces. The normal mode describes a pattern of motions in which all parts of the system move with the same frequency, ω , and in phase. These modes can give insight in the possible movements and regions of flexibility. NMA can be used to approximate the oscillation of an object, thereby describing the motion that has the least inertia. Each mode contains an amplitude, A , describing the extent of movement and a frequency, ω , describing the type of movement. NMA is a powerful method for analysing protein motions and flexibility, especially when alternate crystal structures are available [36] , [37] . Generally, the normal modes responsible for the bulk of the movement are associated with lower frequencies, and it has been shown that in ∼ 50% cases where protein structures in two different conformations have been analysed, their movement could be described by using only one or two low-frequency normal modes [36] , [37] . Normal modes 1–6 correspond to rigid body movements and so are neglected in this analysis. Characterization of the non-zero frequency normal modes (that is, modes ⩾ 7) of the peripheral stalk crystal structures indicates that mode 7 is related to a flexion of the molecule ( Supplementary Movie 10 ) and mode 8 is related to a twisting of the molecule ( Supplementary Movie 11 ). Importantly, the flexion seen in mode 7 and the twisting in mode 8 are in the direction that accommodates the wobbling of the intact complex. Furthermore, combining these two lowest non-zero frequency normal modes shows that PS2 is related to PS1 by movement primarily along these two modes ( Supplementary Fig. S3a ), with flexion of the right-handed coiled-coil tail described by mode 7 ( ω =15.9 cm −1 , A =−124) and twisting by mode 8 ( ω =31.2 cm −1 , A =82). Furthermore, movement of PS2 along these same modes with different amplitudes (mode 7, A =−282; mode 8, A =86) generates a structure similar to PS3 ( Supplementary Fig. S3b ), which is consistent with the EM density of the proximal peripheral stalk. In summary, NMA indicates that the three different conformations of the peripheral stalks can be interconverted using primarily modes 7 and 8. The conformational changes seen between the different crystal structures and NMA independently indicate that the peripheral stalk structure is remarkably flexible in a radial direction and is thus able to accommodate movement towards and away from the central stalk within the intact A-ATPase ( Fig. 4 ). This flexing enables the peripheral stalk to accommodate the radial movement of the catalytic head as the central stalk rotates between different nucleotide states, while still tightly restraining its azimuthal movement and thereby counteracting the torque generated by the rotation of the central stalk. 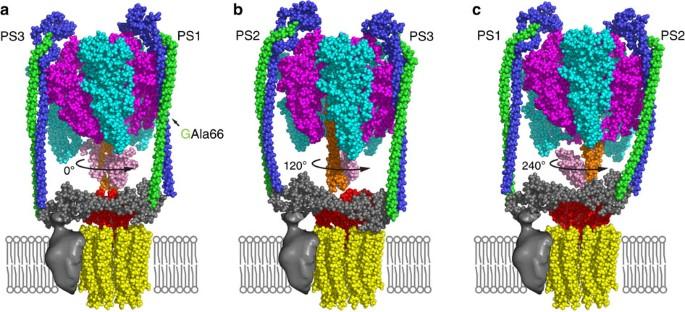Figure 4: Rotating pseudo-atomic model of the A-ATPase with the three peripheral stalks docked at corresponding positions. (a) 0°, (b) 120° and (c) 240° rotation of the central stalk relative to the stator subunits showing how the peripheral stalk dynamics complements the shape of the (AB)3domain during the rotary catalytic cycle. Residue Ala66 of subunit G is highlighted to indicate the transition from hendecad to quindecad repeat in the peripheral stalk. The pdb file for the model shown in (a) is supplied as Supplementary Information. Figure 4: Rotating pseudo-atomic model of the A-ATPase with the three peripheral stalks docked at corresponding positions. ( a ) 0°, ( b ) 120° and ( c ) 240° rotation of the central stalk relative to the stator subunits showing how the peripheral stalk dynamics complements the shape of the (AB) 3 domain during the rotary catalytic cycle. Residue Ala66 of subunit G is highlighted to indicate the transition from hendecad to quindecad repeat in the peripheral stalk. The pdb file for the model shown in ( a ) is supplied as Supplementary Information. Full size image Previously, we speculated that the function of the right-handed coiled-coil present in the peripheral stalk could be to position subunit G in a mechanically superior position during ATP synthesis, in which it would act as an obstruction and restrict bowing of the peripheral stalk during ATP synthesis [26] . However, this does not explain its role during ATP hydrolysis. The analysis of the peripheral stalks presented here provides new insight into the function of the right-handed coiled-coil architecture. The right-handed coiled-coil domain of the peripheral stalk consists of two distinct regions ( Supplementary Fig. S4 ). The N-terminal region is formed by a hendecad (11-mer) repeat leading to a large pitch that results in almost parallel helices. This changes to a quindecad (15-mer) repeat within subunit G at residue Ala66, and consequently the pitch tightens in the C-terminal half of the right-handed coiled-coil where the peripheral stalk comes into contact with subunit B. This tighter coiling towards the C-terminus is further accentuated into a kink in subunit G (reminiscent of an elbow), which brings the C-terminus of subunit G to the opposite side of subunit E relative to the N-terminus. From observation of the differences between the peripheral stalk models ( Fig. 3 ) and the movements of the peripheral stalk with respect to the intact A-ATPase ( Fig. 4 ; Supplementary Movie 9 ), it is clear that this arrangement of a tightening right-handed coiled-coil allows the movement necessary for the accommodation of the wobbling of the catalytic (AB) 3 head. The N-terminal, almost parallel, hendecad repeat region that is not in contact with the (AB) 3 head allows flexing in a purely radial direction, where the inertia would be expected to be least, due to the decreased cross-sectional area (much like the properties of a rectangular beam, Supplementary Fig. S5 ). However, the following quindecad region causes the coil to twist as it flexes owing to its increased pitch in the region of the peripheral stalk that is in contact with subunit B, thus allowing the B-peripheral stalk subunit contacts to remain constant during catalysis, which stabilizes the complex during rotation. The tighter pitch is further increased by the elbow at the C-terminus of subunit G and this allows swivelling (much like the properties of a cardanic pendulum) of the peripheral stalk's head at the top of the complex as the (AB) 3 head wobbles through its catalytic states. The analysis of the F 1 c n crystal structures ( Supplementary Fig. S1 ) and EM class averages [10] , [12] , [17] , [31] shows that the wobbling motion in the A-ATPase is likely to be conserved across all rotary ATPase subtypes, suggesting that peripheral stalks of rotary ATPases across all subtypes and species are likely to undergo a similar flexing/swivelling movement. Indeed, recent work has indicated that the Escherichia coli F-ATPase peripheral stalk is very stiff in an azimuthal direction, at least 10-fold stiffer than its rotor counterpart [38] , which is consistent with the model we propose here. Various structures of F-type ATPases in different catalytic states [28] , [39] , [40] , [41] together with biophysical analysis [38] , [42] clearly indicate that the central rotor of F-type ATPases is highly flexible and can twist along the rotation axis. For A-type ATPases, however, there is not enough structural information available to simulate the dynamics of the central stalk along with the peripheral stalk. While the single peripheral stalk of bacterial F-type ATPases has been predicted to have a right-handed coiled-coil (made of a homodimer of subunit b) [43] , mitochondrial F-type ATPase peripheral stalk subunits show no canonical right-handed coiled-coil repeats. However, despite the lack of sequence homology of A-/V-type and mitochondrial F-type peripheral stalk subunits, the bovine peripheral stalk structure shows features reminiscent of the A-type peripheral stalk overall architecture [25] , [44] . Towards the N-terminus, the alpha helices of subunits b and d run parallel to one another [25] and similarly, like in the A-type peripheral stalk, the pitch decreases towards the C-terminus culminating in a kink of subunit F6 that wraps this subunit around subunit b in a right-handed fashion, reminiscent of an elbow. Again, this will lead to a greater radial flexibility towards the C-terminus of the peripheral stalk to enable accommodation of the wobble of the nucleotide-binding (αβ) 3 complex, while the parallel structure towards the N-terminus retains azimuthal rigidity to counteract rotation. We performed NMA on the crystal structure of the bovine F-ATPase peripheral stalk [25] (pdb 2CLY) to test whether a similar flexibility pattern can be observed. The lowest non-zero frequency modes show that, like its A-type counterpart, the mitochondrial F-type peripheral stalk is indeed most flexible in the radial direction while being rigid in the azimuthal direction. The most divergent feature of F- and A-/V-type ATPase peripheral stalks is the site of attachment of the head of the peripheral stalks to the top of the catalytic domains. Both bacterial and mitochondrial F-ATPases use an additional subunit for this purpose ( δ and the oligomycin sensitivity conferring protein, respectively) and this protein is attached to the central cavity of the (αβ) 3 -ring. This form of attachment is not possible with more than one peripheral stalk per complex and so in A- and V-type ATPases, the peripheral stalks are attached acentrically to the catalytic heads via the globular domain of subunit E. In summary, peripheral stalks from all rotary ATPases may have a conserved architecture that facilitates their function in accommodating the wobbling movement of the catalytic subunits as they progress between different nucleotide states while at the same time restraining their azimuthal movement, thus counteracting the torque of the central rotor. The precise dynamical behaviour of the peripheral stalk needed for its function is built into the structures through the domain architecture of the right-handed coiled-coil and the elbow-hinge region at the interface to the globular domain. In addition, the concerted dynamics of the peripheral stalk in conjunction with the other rotary ATPase subunits ( Supplementary Movie 9 ) provides a possible mechanism for cooperativity within these complexes spanning distances of up to ∼ 250 Å in between ion channel and distal nucleotide-binding subunits. Clearly, more snapshots of intact rotary ATPases are needed at higher resolution to provide a full picture of the dynamics of these molecular rotary machines that incorporate the dynamics of the central stalk and structurally unknown components such as the transmembrane portion of subunit I. Purification of peripheral stalk subunits E and G Crystals containing the full-length subunit G diffracted poorly [26] , and N-terminal sequencing and mass spectrometry of the intact T. thermophilus A-ATPase suggested that subunit G is N-terminally truncated by 17 residues [10] , [18] . The T. thermophilus DNA sequence encoding full-length subunit E and subunit G truncated by its 17 N-terminal residues was cloned into the bicistronic pETDuet-1 vector (Novagen), with subunit G carrying an N-terminal six-histidine tag followed by a tobacco etch virus protease cleavage site. Protein was overexpressed in E. coli BL21 and purified by nickel affinity and gel filtration chromatography as described previously [18] . Crystallization Crystals of the EG peripheral stalk complex were obtained by hanging drop vapour diffusion, in which 1 μl drops of 3 mg ml −1 protein solution were mixed with 1 μl drops of crystallization buffer containing 100 mM HEPES (pH 7.5), 200 mM calcium acetate and 40% (v/v) PEG 400, and equilibrated in Linbro plates (Hampton Research, Aliso Viejo, CA, USA) at 20 °C. Small needles were obtained after 48 h with the longest dimension in the order of 100 μm belonging to space group P2 1 2 1 2 with two EG heterodimers in the asymmetric unit. Crystals were mounted in loops and flash frozen in liquid nitrogen. Preparation of heavy-atom derivatives Derivatives were obtained by soaking single crystals for 10 min in crystallization buffer supplemented with 100 mM of either Dysprosium(III) chloride or Lutetium(III) acetate (Hampton Research) followed by washing in crystallization solution to remove excess heavy atoms. Data collection and structure determination A 2.25-Å resolution native data set was obtained at beamline ID14-4 at the European Synchrotron Radiation Facility, Grenoble, France, and SAD data sets of the derivatives were obtained using beamline MX-2 at the Australian Synchrotron, Melbourne, Australia. Data sets with high redundancy were collected for each crystal, and were indexed and integrated using Mosflm [45] or XDS [46] , and scaled with SCALA [47] . The native data set showed strong anisotropy and was truncated in the a* direction to 2.5-Å resolution using the UCLA MBI–Diffraction Anisotropy Server [48] , phases were obtained via MIRAS using data sets of Lutetium- and Dysprosium-soaked crystals. AUTOsharp [49] was used with two heavy-atom sites for each data set and optimized solvent flattening/flipping using SOLOMON. The phases obtained from SOLOMON were combined with the native data set and used to build an initial atomic model using autoBuild in PHENIX [50] . This model was then subjected to iterative cycles of refinement using PHENIX [50] and Refmac 5 [51] with TLS [52] , and rebuilding using COOT [53] , with guidance from MolProbity [54] to identify errors in the model. A final model was produced with a crystallographic R-factor of 22.3% (Rfree 26.3%), with a MolProbity score of 1.72 (96th percentile) and 0.2% Ramachandran outliers. Table 2 gives the crystallographic statistics for all three data sets and Supplementary Fig. S6 shows an example of the refined electron density map. Structure analyses MDFF was set up using the MDFF package in VMD [55] and performed using NAMD [34] . Each structure was rigid body docked into the proximal EM density using the UCSF Chimera package [35] , and subsequently placed in a neutrally charged water box with 20-Å padding. The EM density was converted into MDFF potential and a simulation was run until convergence was achieved ( ∼ 200 ps). NMA was performed using the elNémo web server [36] , which computes the low-frequency normal modes for a given protein structure in PDB format. Superpositions were performed with SUPERPOSE within the CCP4 programme suite [56] . Vectors were obtained via CCP4mg [57] . Geometric analysis of the vectors, as shown in Table 1 , was performed by calculating the arccosine of the dot products of the central axes through the proteolipid rings and the rings formed by the nucleotide-binding subunits. Morphs and movies Morphs were produced using the UCSF Chimera package [35] from the Resource for Biocomputing, Visualization, and Informatics at the University of California, San Francisco (supported by NIH P41 RR001081). Images and movies were made using the PyMOL Molecular Graphics System, Version 1.3, Schrödinger, LLC and CCP4mg [57] . Accession codes: Atomic coordinates and structure factors for the 2.25-Å resolution peripheral stalk crystal structure have been deposited in the Protein Data Bank under accession code 3V6I . How to cite this article: Stewart, A. G. et al . The dynamic stator stalk of rotary ATPases. Nat. Commun. 3:687 doi: 10.1038/ncomms1693 (2012).